Experimental magic state distillation for fault-tolerant quantum computing Any physical quantum device for quantum information processing (QIP) is subject to errors in implementation. In order to be reliable and efficient, quantum computers will need error-correcting or error-avoiding methods. Fault-tolerance achieved through quantum error correction will be an integral part of quantum computers. Of the many methods that have been discovered to implement it, a highly successful approach has been to use transversal gates and specific initial states. A critical element for its implementation is the availability of high-fidelity initial states, such as |0〉 and the 'magic state'. Here, we report an experiment, performed in a nuclear magnetic resonance (NMR) quantum processor, showing sufficient quantum control to improve the fidelity of imperfect initial magic states by distilling five of them into one with higher fidelity. Quantum information processing (QIP) [1] , [2] , [3] , [4] promises a dramatic computational speed-up over classical computers for certain problems. In implementation, the physical quantum devices for QIP are subject to errors owing to the effects of unwanted interactions with the environment or quantum control imperfections. In order to be reliable and efficient, quantum computers will need error-correcting or error-avoiding methods. One method to achieve fault-tolerant quantum computation is to encode the state of a single quantum bit (qubit) into blocks of several qubits that are more robust to errors. On the basis of this idea, quantum error correction codes, the theory of fault-tolerant quantum computation and the accuracy threshold theorem have been developed [5] , [6] , [7] . A key element for fault-tolerant quantum computation is to avoid bad error propagation. One straightforward protocol is to use transversal gates where an error occurring on the k th qubit in one block can only propagate to the k th qubit in the other blocks. A highly successful approach to achieve fault-tolerant universal quantum computation is based on quantum error correcting codes, with gates from the Clifford group that can be applied transversally [8] , [9] . Unfortunately, they are not universal [10] , [11] and they must be supplemented with the preparation of not only the |0〉 state but also another type of state such as a 'magic state' [12] , [13] , [14] , [15] , [16] . Thus, a critical element for fault-tolerance is the availability of high-fidelity magic states. Consequently, in the pursuit of experimental fault-tolerant quantum computation, it is important to determine whether we have sufficient experimental control to prepare these magic states. In general, these will be prepared with some imprecision. The states can be improved by distilling many magic states to produce a fewer number of them which have higher fidelity. Here, we report an experiment, performed in a seven-qubit nuclear magnetic resonance (NMR) quantum processor, showing sufficient quantum control to implement a distillation protocol based on the five-bit quantum error correcting code [12] , [17] that uses only Clifford gates. The fidelity of imperfect initial magic states is improved by distilling five of them into one with higher fidelity. Theoretical protocol The Clifford group is defined as the group of operators that maps the Pauli group onto itself under conjugation. The Pauli group is defined as [1] where σ x , σ y , σ z , and denote the Pauli matrices and identity operator, respectively. The Clifford group on n qubits is a finite subgroup of the unitary group U (2 n ) and can be generated by the Hadamard gate H , the phase-shift gate S ph , and the controlled-not gate CNOT represented as in the computational basis {|0〉, |1〉}. An arbitrary one-qubit state can be represented in the Bloch sphere as where p x , p y and p z are the three polarization components of the state. The magic states [12] are defined as the 8 states with , , ( T -type) and the 12 states with p x =0, , ; p y =0, , ; p z =0, , ( H -type). These states are called 'magic' because of their ability, with Clifford gates, to enable universal quantum computation and the ability to be purified, when it has been prepared imperfectly, using only Clifford group operations [12] . In our current work, we distill an imperfect magic state into a T -type magic state represented as To quantify how near a state ρ is to the magic state, we define the m-polarization (polarization in the direction of the magic state) The distillation algorithm requires five copies of a faulty magic state ρ in = ρ ⊗ 5 as the input state. In the original proposal [12] , the measurement of four stabilizers S i ( i =1, ..., 4) is applied to ρ in , where , , and . If the outcome of any of these observables is −1, the state is discarded and the distillation fails. If the results of all the measurement are +1, corresponding to the trivial syndrome, one applies the decoding transformation for the five-qubit error-correcting code [17] to the measured state and obtains the output state ρ dis ⊗ |0000〉〈0000| where ρ dis has the output m-polarization p out . If the input m-polarization distillation is possible and p out > p in and produces a state nearer to the magic one. In an iterative manner, it is possible to obtain the output m-polarization approaching 1. As NMR QIP is implemented in an ensemble of spin systems, only the output of expectation values of ensemble measurements [18] are available. Consequently, the above projective measurement of the stabilizers cannot be implemented in our experiment. However, as the decoding operation is just a basis transformation from one stabilizer subspace to another, it is possible to evaluate the result of the distillation after decoding. Therefore, we directly apply the decoding operation to the input state ρ in , and the output state becomes a statistical mixture of 16 possible outcomes represented as where θ i is the probability of each outcome, and | i 〉=|0000〉, |0001〉, ..., |1111〉, for i =0, 1, 2, ..., 15, noting ρ 0 = ρ dis . Now measuring |0〉 on all four qubits in | i 〉 indicates a successful purification. We can obtain θ i and ρ i using partial quantum state tomography [19] . Experimental results The data were taken with a Bruker 700 MHz spectrometer. We choose 13 C-labelled trans-crotonic acid dissolved in d6-acetone as a seven-qubit register. 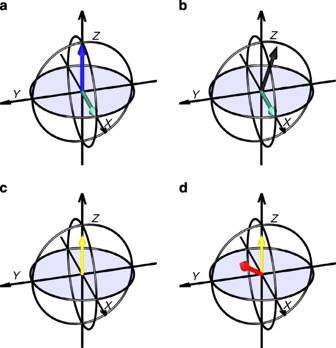Figure 1: The evolution ofσσσΣρzin the preparation of a faulty magic state in Bloch sphere. Arrows represent the states of the qubit. (a) Aπ/2 rotation alongyaxis transformsσz(blue) toσx(green). (b) Anotherπ/2 rotation along direction [cosa, sina, 0] transformsσx(green) toσxcos2a+σycosasina−σzsina(black). In phase cycling, we apply the secondπ/2 rotation by changingatoπ+ato transformσxtoσxcos2a+σycosasina+σzsina. After taking the average of thexandycomponents to zero, the polarization is reduced to −σzsina, shown as the yellow arrow in (c), noting thata∈[π, 3π/2]. (d) A final rotation with angle arccosalongtransforms −σzsina(yellow) to(red). The structure of the molecule and the parameters of qubits are shown in Table 1 . We prepare a labelled pseudo-pure state ρ s = 00 σ z 0000 using the method in ref. 20 , where 0 =|0〉〈0| and the order of qubits is M, H 1 , H 2 , C 1 , C 2 , C 3 , C 4 . One should note that we are using the deviation density matrix formalism. Table 1 Characteristics of the molecule trans-crotonic acid. Full size table We prepare an initial imperfect magic state with three equal polarization components by depolarizing the state First, we apply a π /2 pulse to rotate the state 0 to and then another π /2 pulse along direction [cos a , sin a , 0] is applied. We use phase cycling to average the x and y components of the state to zero, and therefore the polarization of the spin initially in the state 0 is reduced. The depolarized state is represented as Finally, we apply a rotation with angle arccos about the direction to obtain an imperfect magic state where p =−sin a . The evolution of σ z in the preparing ρ is shown in Figure 1 . By doing the above operation for qubits M, C 1 , C 2 , C 3 , C 4 , respectively, we obtain five copies of the imperfect magic states ρ in = ρ ⊗ 5 . Exploiting partial state tomography, we measure p for each qubit and use the average as the input m-polarization p in for ρ in . Figure 1: The evolution of σσσΣρ z in the preparation of a faulty magic state in Bloch sphere. Arrows represent the states of the qubit. ( a ) A π /2 rotation along y axis transforms σ z (blue) to σ x (green). ( b ) Another π /2 rotation along direction [cos a , sin a , 0] transforms σ x (green) to σ x cos 2 a + σ y cos a sin a−σ z sin a (black). In phase cycling, we apply the second π /2 rotation by changing a to π + a to transform σ x to σ x cos 2 a + σ y cos a sin a+σ z sin a . After taking the average of the x and y components to zero, the polarization is reduced to − σ z sin a , shown as the yellow arrow in ( c ), noting that a ∈ [ π , 3 π /2]. ( d ) A final rotation with angle arccos along transforms − σ z sin a (yellow) to (red). 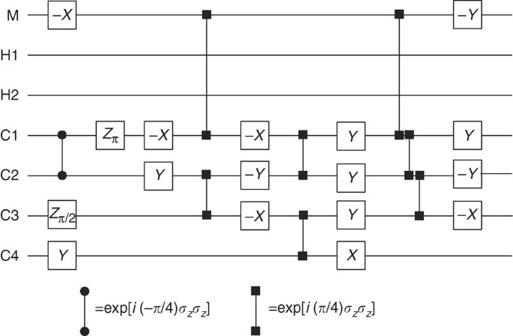Figure 2: Gate sequence for magic state distillation. The sequence is constructed from the five qubit error correction code17, where ±X=exp(±iπσx/4), ±Y=exp(±iπσy/4) and ±Zα=exp(−iασz/2). Qubits labelled as M, C1, C2, C3and C4are used to encode the five copies of the initial state. Owing to the nature of the algorithm, the carbon C1contains the distilled magic state only when M, C2, C3and C4are in the |0000〉 state. It is important to emphasize that all gates are Clifford gates. The refocussing pulses (which also decouple H1and H2) are not shown. Full size image The circuit for the distillation operation is shown in Figure 2 . C 1 carries the distilled state after the distillation. With partial state tomography, we can determine θ i and ρ i in equation (5), where ρ 0 = ρ dis , from which the output m-polarization p out is obtained. 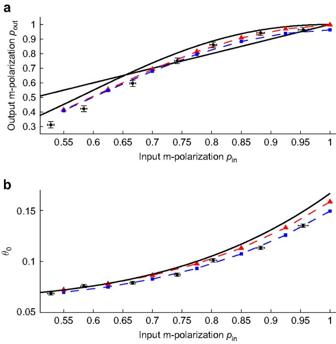Figure 3: Experimental results after the completion of magic state distillation. Output m-polarization of the faulty magic state (a) and the probabilityθ0(b) of finding this state in the mixture of outcomes (see equation (5)) as a function of the input m-polarization of the initial faulty magic state. The experimental data are represented by the filled circles and the error bars are estimated from the uncertainty of the fitting parameters. The line inarepresents the functionpout=pin. The experimental points above the line show the states that have been distilled, whereas the points below the line show the states that cannot be distilled in the protocol. The theoretical prediction is represented by the black solid curves. The blue squares and red triangles, connected by dashed lines for visual convenience, are the simulation results where the dephasing rates are chosen asT2*andT2(Figure 1), respectively. The effectiveT2during the experiment should be similar to the Hahn echoT2. The deviation can be attributed to other error sources (see text). The dephasing times of H1and H2actually do not influence the results because H1and H2can be effectively assumed in0andσzduring the whole experiment, respectively. The experimental results for magic state distillation for various p in are shown in Figure 3 , where a and b show the measured p out and θ 0 , respectively. The straight line in a represents the function p out = p in . The data points above the line show the states that have been distilled experimentally. Figure 2: Gate sequence for magic state distillation. The sequence is constructed from the five qubit error correction code [17] , where ± X =exp(± iπσ x /4), ± Y =exp(± iπσ y /4) and ± Z α =exp(− iασ z /2). Qubits labelled as M, C 1 , C 2 , C 3 and C 4 are used to encode the five copies of the initial state. Owing to the nature of the algorithm, the carbon C 1 contains the distilled magic state only when M, C 2 , C 3 and C 4 are in the |0000〉 state. It is important to emphasize that all gates are Clifford gates. The refocussing pulses (which also decouple H 1 and H 2 ) are not shown. Full size image Figure 3: Experimental results after the completion of magic state distillation. Output m-polarization of the faulty magic state ( a ) and the probability θ 0 ( b ) of finding this state in the mixture of outcomes (see equation (5)) as a function of the input m-polarization of the initial faulty magic state. The experimental data are represented by the filled circles and the error bars are estimated from the uncertainty of the fitting parameters. The line in a represents the function p out = p in . The experimental points above the line show the states that have been distilled, whereas the points below the line show the states that cannot be distilled in the protocol. The theoretical prediction is represented by the black solid curves. The blue squares and red triangles, connected by dashed lines for visual convenience, are the simulation results where the dephasing rates are chosen as T 2 * and T 2 ( Figure 1 ), respectively. The effective T 2 during the experiment should be similar to the Hahn echo T 2 . The deviation can be attributed to other error sources (see text). The dephasing times of H 1 and H 2 actually do not influence the results because H 1 and H 2 can be effectively assumed in 0 and σ z during the whole experiment, respectively. Full size image The implementation time of the distillation procedure is about 0.1 s, a non-negligible amount of time (10%) compared with coherence time ( T 2 in Table 1 ). Hence, the decay of the signals due to the limitation of coherence time is an important source of errors. We extract p out by measuring the ratio of θ 0 p out and θ 0 , where these two factors are obtained by various single coherent terms in a series of experiments. We have assumed that the terms have the same amount of decoherence. The results of simulations with dephasing rates T 2 * and T 2 are shown in Figure 3 as blue squares and red triangles. The simulation results show that the decoherence rates are long enough to allow the distillation and suggest that the deviation of θ 0 from the theoretical expectation can be mainly attributed to relaxation effects. Additionally, imperfection in the shaped pulses and inhomogeneities of magnetic fields also contribute to errors. We modify the original distillation protocol by avoiding the projective measurement, which is not possible to implement in the NMR QIP's. We exploit partial state tomography to obtain each output in the mixture of the outcomes after the distillation, and only in a post-processing step do we choose the one we need. Although we could access the |0000〉〈0000| subspace using a procedure similar to the pseudo-pure state preparation, the method would take substantially longer time and would be more error-prone. In this work, we aim for a quantitative result, that is, increasing the magic state purity. We need to minimize the readout manipulations to avoid control-error-induced distortions of the inferred final state and associated purity. Hence, we limited ourselves to simple high-fidelity readout procedures. In summary, we have implemented a protocol for distilling magic states on the basis of the five qubit quantum error correction code. We exploit five qubits by controlling a seven-qubit NMR quantum information processor. The experiment shows that we have obtained enough control to purify faulty magic states through distillation. Overview of the experiment To implement the experiment, we exploit standard Isech and Hermite-shaped pulses as well as numerically optimized GRAPE pulses [21] to implement single-spin operations. The GRAPE pulses are optimized to be robust to radio frequency (r.f.) inhomogeneities and chemical shift variations. All pulses are combined in a custom-built software compiler [22] . The compiler loads the information about the internal Hamiltonian and the desired unitary transformation from simple predefined building blocks. The blocks are then systematically put together to form a pulse sequence, ensuring that the errors in the building blocks do not propagate as the sequence progresses. R.f. selection The effect of pulse imperfections because of r.f. inhomogeneities is reduced by selecting signal based on r.f. power [20] . The signal selection is achieved by spatially selecting molecules from a small region in the sample. The method is similar to imaging methods [23] and has been used in previous works [20] . Here, we substitute the original pulse sequence proposed in ref. 20 by a single GRAPE pulse to optimize the performance. Besides reducing r.f inhomogeneities, the spatial selection of spins can also reduce the static field inhomogeneities and therefore reduces the loss of signal during the experiment [24] . We have found that the effective relaxation time ( T 2 * ) of spins after the r.f. selection increases significantly, for example, up to a factor 2 for some spins. 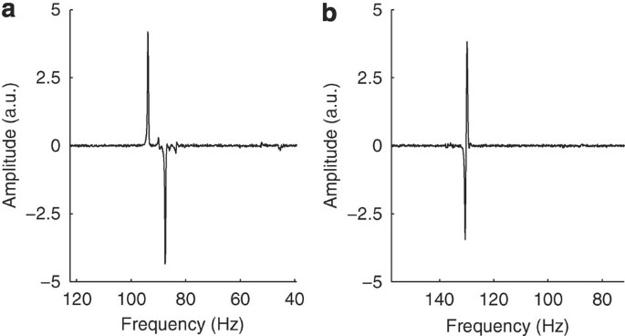Figure 4: Pseudo-pure state NMR spectra. (a,b) Spectra of C1and C2obtained byπ/2 readout pulses when the system lies in the labelled pseudo-pure stateρs=00σz0000. The vertical axes have arbitrary but the same units. Partial state tomography We use the spectra obtained from the labelled pseudo-pure state ρ s = 00 σ z 0000 shown in Figure 4 as a phase reference and to normalize the signals in C 1 and C 2 spectra, for measuring the initial and output m-polarization. To obtain the reduced density matrix of C 1 through the partial state tomography, we expand equation (5) as a sum of product operators [19] , and represent ρ i as Figure 4: Pseudo-pure state NMR spectra. ( a , b ) Spectra of C 1 and C 2 obtained by π /2 readout pulses when the system lies in the labelled pseudo-pure state ρ s = 00 σ z 0000 . The vertical axes have arbitrary but the same units. Full size image In the expansion, there are 128 terms that are required to be determined by the experiment. The coefficients of such expansion can be directly related to the measurable spectral amplitudes [19] . On the other hand, such coefficients can also be related to the relevant parameters of equation (5), that is, p i,x , p i,y , p i,z and θ i for i =0, 1, 2, ..., 15. The relation between these parameters and the NMR observables can be expressed by the set of linear equations The n th element, C ( n ), of the column vector C is the coefficient related to the operator with the order of qubits M, H 1 , H 2 , C 1 , C 2 , C 3 , C 4 , where s can be one element of the Pauli group { σ x , σ y , σ z I } and the vector is the four digit binary representation of the integer n −1. For s=σ x , σ y , σ z and I , R ( n )= θ n p n , x , θ n p n , y , θ n p n , z and θ n , respectively. The elements of the matrix A are given by Providing that we have all necessary coefficients measured, we can reconstruct the distilled states using the following approach. First, we fit the NMR spectral lines to the yield complex amplitudes for measuring all necessary coefficients [19] . 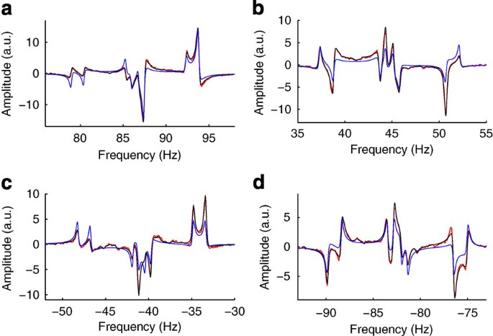Figure 5: Spectrum of C1after the completion of distillation forpin=0.95. The spectra are divided in four different parts shown as (a–d) for better visualization. The vertical axes have arbitrary but the same units. The experimentally measured, fitting and ideal spectra are shown as the red, black and blue curves, respectively. Figure 5 illustrates the spectra of C 1 after the completion of distillation for p in =0.95, where the experimentally measured, fitted and ideal spectra are shown as the red, black and blue curves, respectively. Then the state (equation (5)) is reconstructed by solving the set of equation (9). Our calculation shows that four readout operations are sufficient to determine all coefficients: first, read out on C 1 ; second, read out on C 1 after the application of a π /2 pulse; third, read out on C 2 after the application of a π /2 pulse; and forth, read out on C 2 after a polarization transfer from H 1 to C 2 . The last two readout operations are sufficient to measure all θ i , and the first two are used to measure θ i ρ i . The errors for the coefficients, as well errors for p i,x , p i,y and p i,z and θ i , are estimated from the uncertainty of the fitting parameters. The measured initial and output m-polarization, as well as θ i and ρ i , are listed in Supplementary Tables S1–S10 . The comparison of the various measured ρ 0 with the theory is shown as equations (1,2,3,4,5,6,7) in the Supplementary Methods . Figure 5: Spectrum of C 1 after the completion of distillation for p in =0.95. The spectra are divided in four different parts shown as ( a – d ) for better visualization. The vertical axes have arbitrary but the same units. The experimentally measured, fitting and ideal spectra are shown as the red, black and blue curves, respectively. Full size image How to cite this article: Souza, A. M. et al . Experimental magic state distillation for fault-tolerant quantum computing. Nat. Commun. 2:169 doi: 10.1038/ncomms1166 (2011).